Plasmonic substrates for multiplexed protein microarrays with femtomolar sensitivity and broad dynamic range Protein chips are widely used for high-throughput proteomic analysis, but to date, the low sensitivity and narrow dynamic range have limited their capabilities in diagnostics and proteomics. Here we present protein microarrays on a novel nanostructured, plasmonic gold film with near-infrared fluorescence enhancement of up to 100-fold, extending the dynamic range of protein detection by three orders of magnitude towards the fM regime. We employ plasmonic protein microarrays for the early detection of a cancer biomarker, carcinoembryonic antigen, in the sera of mice bearing a xenograft tumour model. Further, we demonstrate a multiplexed autoantigen array for human autoantibodies implicated in a range of autoimmune diseases with superior signal-to-noise ratios and broader dynamic range compared with commercial nitrocellulose and glass substrates. The high sensitivity, broad dynamic range and easy adaptability of plasmonic protein chips presents new opportunities in proteomic research and diagnostics applications. Protein microarray chips have found numerous applications in expression profiling, drug–target binding assays, and high-throughput proteomics [1] , [2] . To date, only a few reports exist detailing the use of conventional, planar protein microarrays in biomarker detection assays for disease diagnosis and monitoring [3] , [4] . Although microarray assays facilitate high-throughput protein analysis with low sample volume requirements, thus far, the methodology affords little improvement of detection limits or dynamic range compared with enzyme-linked immunosorbent assays (ELISAs). Several creative methods for improving the sensitivity and detection limits of protein microarray sandwich assays have been devised [5] , [6] , [7] , [8] . While promising for early disease detection applications, when serum biomarkers are extremely dilute [8] , [9] , these methods require extra assay steps, complex assay preparation, non-traditional data-processing, and/or specialized signal quantification apparatus, such as micro-Raman scattering instrumentation [5] . Metal-enhancement of fluorescence is an attractive alternative to complex amplification strategies in bioassays [5] , [10] , [11] . Appropriate fluorophores positioned close to roughened or nanoscopic noble metallic surfaces may undergo an increase in emission intensity leading to improved signal-to-noise ratios [12] , [13] . Experiments using fluorescently-labelled antibodies in proximity to silver-island films [14] , and deposited gold nanoparticles [15] have demonstrated the potential for improving signal-to-noise ratios in protein assay measurements with enhancement factors of 10–40-fold [10] . However, to date, fluorescence enhanced multiplexed microarray assays have not been demonstrated, and sensitive and quantitative measurements of disease biomarkers have been hampered by the inability to produce fluorescence-enhancing substrates that are uniform over large areas and stable over time [16] . Here we present protein microarrays on plasmonic gold substrates, enabling multiplexed protein assays affording detection limits as low as a few fM, with six orders of magnitude dynamic range, for the first time. A nanostructured gold film prepared by uniform, solution-phase growth onto whole glass slides affords near-infrared fluorescence enhancement (NIR-FE) of up to 100-fold, useful for significant improvement of protein microarray detection assays. We demonstrate that the resulting microarray substrates (μArray/Au) are compatible with standard microarray scanners and afford highly sensitive measurements over a broad dynamic range of a model cancer biomarker, carcinoembryonic antigen (CEA). Compared with standard glass-supported microarrays, our μArray/Au affords an expansion of dynamic range of protein microarrays by up to three orders of magnitude. The femtomolar detection limit and broad dynamic range afforded by μArray/Au allow for quantification and monitoring of CEA in serum samples of mice during the early-stage growth of xenograft LS174T tumours, opening the possibility of NIR-FE protein microarrays for early disease detection and therapeutic monitoring. Finally, the broadened dynamic range afforded by μArray/Au is employed for multiplexed detection of human autoantibodies, demonstrating the potential for NIR-FE protein microarrays to serve not only as sensitive diagnostic assays, but also as tools to expand the capabilities of proteomic research into the pathogenesis and pathophysiology of disease states. Optimization for near-infrared fluorescence enhancement Gold-on-gold films (Au/Au, referring to Au seeding followed by Au growth) were prepared on standard glass slides by a simple seeding and growth process in solution phase [17] , [18] , [19] (Methods), producing elongated, tortuous nanoscale gold islands ( Fig. 1a ) on glass with plasmon resonances in the near-infrared ( Fig. 1b ). The gold-seeding step was optimized to yield a dense and uniform distribution of Au nanoparticles on the substrate, and variation of the selective gold-growth condition onto the gold seeds resulted in Au/Au films with a range of plasmonic resonances exhibiting monotonic red-shifting and increasing film thickness with increasing gold precursor concentrations ( Supplementary Fig. S1 ). Increasing Au/Au film thickness was accompanied by increasing gold island sizes and reduction in the density of inter-island gaps, followed by eventual coalescence of the gold islands into a continuous film ( Supplementary Fig. S2 ) [17] . 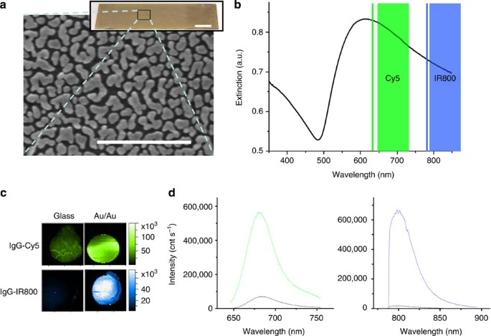Figure 1: Plasmonic gold-on-gold nano-island films enhance the fluorescence of near-infrared fluorophores. (a) Scanning electron micrograph (scale bar, 1 μm) of a solution-phase grown Au/Au film on glass showing the nanoscopic gold island morphology. Inset shows digital photograph of an Au/Au film-coated glass slide with scale bar, 1 cm. (b) Extinction spectrum of Au/Au film overlaid with the excitation (line) and emission (shaded area) regions of Cy5 and IR800 dyes, respectively. (c) Fluorescence intensity maps of IgG–Cy5 (top) and IgG-IR800 (bottom) conjugates drop dried onto glass or the Au/Au film from (a). Images for each fluorophore on glass and Au/Au are shown on the same intensity scale for comparison. Analyte spot size is∼2 mm in diameter. (d) Fluorescence emission spectra of IgG-bound Cy5 (left) and IR800 (right) dried onto the Au/Au film (shown in green and blue, respectively) from (a) as well as glass for comparison (shown in black). Figure 1: Plasmonic gold-on-gold nano-island films enhance the fluorescence of near-infrared fluorophores. ( a ) Scanning electron micrograph (scale bar, 1 μm) of a solution-phase grown Au/Au film on glass showing the nanoscopic gold island morphology. Inset shows digital photograph of an Au/Au film-coated glass slide with scale bar, 1 cm. ( b ) Extinction spectrum of Au/Au film overlaid with the excitation (line) and emission (shaded area) regions of Cy5 and IR800 dyes, respectively. ( c ) Fluorescence intensity maps of IgG–Cy5 (top) and IgG-IR800 (bottom) conjugates drop dried onto glass or the Au/Au film from ( a ). Images for each fluorophore on glass and Au/Au are shown on the same intensity scale for comparison. Analyte spot size is ∼ 2 mm in diameter. ( d ) Fluorescence emission spectra of IgG-bound Cy5 (left) and IR800 (right) dried onto the Au/Au film (shown in green and blue, respectively) from ( a ) as well as glass for comparison (shown in black). Full size image Enhanced fluorescence of fluorophores on Au/Au films was first gleaned by drop drying immunoglobulin G molecules (IgGs) conjugated to the near-infrared fluorescent dyes cyanine-5 (Cy5) and IR800 onto Au/Au films of various thicknesses, with a range of optical extinction maxima, as well as onto a bare glass slide. Integration of fluorescence resulted in a range of observed relative enhancement factors compared with the glass substrate, initially increasing with increasing film thickness to a maximum, followed by a decrease ( Fig. 1c ; Supplementary Fig. S3 ). The ensemble fluorescence intensity probably reflects both quenching and enhancement effects, and it was experimentally determined that within the separation distance to the plasmonic film ( ∼ 0–10 nm) provided by the size of the IgG molecule, Cy5 was maximally enhanced ( ∼ 3-fold) by Au/Au films with a plasmon resonance peak of 575 nm whereas IR800 was maximally enhanced ( ∼ 17-fold) by a slightly thicker film with a plasmon resonance peak of 610 nm ( Fig. 1d ). Aside from intensification, the emission maxima and spectral shape of both Cy5 and IR800 are unchanged during enhancement. Direct microarray printing of serially diluted dye-labelled-IgGs onto optimized Au/Au films or glass slides revealed not only enhanced fluorescence intensity, but also a broadened dynamic range of detectable protein concentrations on Au/Au substrates over glass ( Supplementary Fig. S4 ). NIR-FE protein microarray assays on Au/Au films With Au/Au film parameters optimized for NIR-FE of Cy5 and IR800, protein microarrays on Au/Au films (μArray/Au) were prepared by modifying the surface of the gold film with branched poly(ethylene glycol)-carboxylate (PEG-carboxylate), covalently conjugated to a thiol-containing cysteamine self-assembled monolayer (Methods) [5] . This surface modification increases the hydrophilicity of the gold island film and reduces nonspecific interaction of proteins with the gold surface while providing covalent coupling points for proteins via amidation. Monoclonal mouse anti-CEA IgG was deposited robotically onto N-hydroxysuccinimide-activated PEG-carboxylate-coated Au/Au films, and on glass slides for comparison, by solid-pin contact printing at 5 μM (concentrations below 5 μM typically gave lower assay intensities, Supplementary Fig. S5 ) in microarray format. Following a blocking step, CEA-spiked into pure fetal bovine serum was incubated above the mouse anti-CEA array features at concentrations ranging from 100 pM to 1 fM (1 fM=0.2 pg ml −1 ) along with a serum-only blank (Methods). Detection by polyclonal rabbit anti-CEA IgG and subsequent labelling by goat anti-rabbit IgG conjugated to IR800 ( Supplementary Fig. S6 ) demonstrated sensitivity over six orders of magnitude, down to a detection limit of ∼ 5 fM ( Fig. 2 ), defined as blank plus three standard deviations (that is, the standard error of the means of duplicate blank assay features). The resulting μArray/Au assay afforded a relative fluorescence enhancement of IR800 by up to ∼ 100-fold compared with microarrays on glass substrates ( Fig. 2b ). 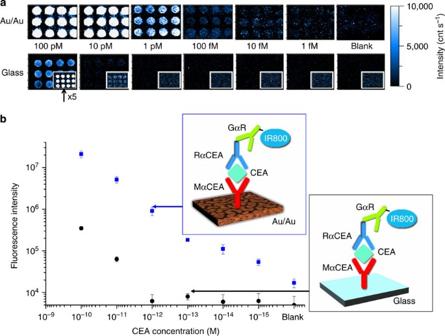Figure 2: Near-infrared fluorescence enhanced protein microarrays on gold substrates probed by IR800. (a) Top panel: μArray/Au fluorescence maps generated by integration of goat anti-rabbit IgG-IR800 fluorescence emission at 785 nm excitation for different concentrations (12 duplicate spots for each concentration) of the analyte, CEA spiked into whole, undiluted serum. Lower panel: fluorescence maps on the same intensity scale as the top panel for comparison, generated in an identical fashion on a glass substrate (inset shows fluorescence maps with intensity increased by ×5). (b) Calibration curves for CEA quantification were generated by averaging the integrated fluorescence intensity of goat anti-rabbit IgG-IR800 emission over the 12 duplicate microarray spots for each CEA concentration on a μArray/Au assay as well as a protein microarray on glass as shown in schematics. Error bars represent the standard deviation of the mean over the 12 duplicate assay features. Figure 2: Near-infrared fluorescence enhanced protein microarrays on gold substrates probed by IR800. ( a ) Top panel: μArray/Au fluorescence maps generated by integration of goat anti-rabbit IgG-IR800 fluorescence emission at 785 nm excitation for different concentrations (12 duplicate spots for each concentration) of the analyte, CEA spiked into whole, undiluted serum. Lower panel: fluorescence maps on the same intensity scale as the top panel for comparison, generated in an identical fashion on a glass substrate (inset shows fluorescence maps with intensity increased by ×5). ( b ) Calibration curves for CEA quantification were generated by averaging the integrated fluorescence intensity of goat anti-rabbit IgG-IR800 emission over the 12 duplicate microarray spots for each CEA concentration on a μArray/Au assay as well as a protein microarray on glass as shown in schematics. Error bars represent the standard deviation of the mean over the 12 duplicate assay features. Full size image Identical CEA sandwich assays performed on branched PEG-carboxylate-modified glass slides and commercially available epoxide-functionalized glass slides ( Supplementary Fig. S7 ) showed slightly worse assay performance than unfunctionalized Superfrost Plus glass slides. All of the microarrays processed on glass substrates, commercial or home-made, with various surface functionalization, were found inferior to μArray/Au, indicating that NIR-FE, and not surface chemistry, was the major cause of improved signal-to-noise and dynamic range of μArray/Au protein assays. The ∼ 100-fold increase in signal-to-noise afforded by μArray/Au improved the sensitivity of CEA detection in full serum by ∼ 5,000-fold relative to the glass substrate and afforded a broadened dynamic range of 6 orders of magnitude ( Fig. 2 ). In addition to IR800, Cy5-labelled μArray/Au assays also demonstrated relative fluorescence enhancements of ∼ 15-fold ( Supplementary Fig. S8 ), affording a similar dynamic range and detection limit of CEA as the IR800-labelled μArray/Au assay. Exploring the origins of NIR-FE from μArray/Au We investigated the origins of the observed increase in fluorescence intensity of both Cy5 and IR800 fluorophores on μArray/Au assays compared with those on glass. Sandwich assays, including protein microarrays, are inherently dependent on the quantity of antibody (or capture species) immobilized onto the substrate. Scanning electron microscope (SEM) imaging revealed that the nano-island structure of Au/Au films afforded a ∼ 70% increase in surface area compared with glass slides ( Supplementary Fig. S9 ), an insufficient difference to account for observed fluorescence enhancements from 15- to 100-fold. We note that our nanostructured Au/Au films are unique over vapour phase deposited continuous Au films in affording high fluorescence enhancement. On continuous gold films, prepared by high-vacuum electron beam evaporation methods, we found that fluorescence quenching, rather than enhancement was observed when protein sandwich assay experiments were performed ( Supplementary Fig. S10 ). Au/Au film plasmon resonance, gold island size and shape, and inter-island gap spacing were important variables in obtaining optimal fluorescence enhancement in protein microarray assays. SEM imaging revealed that Au/Au films optimal for NIR-FE possessed elongated gold nanoparticle islands with area ∼ 14,000±11,500 nm 2 , and small inter-island gap distances of 36±23 nm, resulting in a broad surface plasmon resonance extending into the near-infrared. The necessity for optimal nanoscopic gold island sizes and small inter-island gaps is exemplified by the fact that thin Au/Au films containing small ( ∼ 2,200±1,700 nm 2 ) gold islands ( Supplementary Fig. S2a ), or thicker, semi-continuous (Au island size ∼ 38,500±20,000 nm 2 , Supplementary Fig. S2c ) and continuous ( Supplementary Fig. S2d ) Au/Au films afforded little or no fluorescence enhancement for μArray/Au assays. The abundant nanoscale gaps in our optimal Au/Au films ( Supplementary Fig. S2b ) could afford enhancement of local excitation electric fields, leading to increased excitation rates of fluorophores, thus contributing to the observed fluorescence enhancement in our microarrays [20] , [21] . We also measured the excited state lifetimes for fluorophores used in our μArray/Au sandwich assays by time-correlated single photon counting (Methods). The quantum yield ( η ) of a fluorophore is defined by the ratio of the radiative decay rate ( k rad ) to the total excited state decay rate, η = k rad /( k rad + k nr ), where k nr is the non-radiative decay rate. Cy5-labelled CEA sandwich assays were used to probe the excited state lifetime of Cy5 on Au/Au films as well as on glass ( Fig. 3 ). A clear reduction in lifetime was observed, with the Cy5 fluorescence lifetime reduced to 0.32 nsec on a μArray/Au assay compared with its longer free space value of ∼ 1.5 nsec (ref. 22 ). It is possible that both electric field enhancement and increased radiative decay rate due to fluorophore coupling to the dipolar plasmonic modes in the underlying Au/Au film contributed to the observed increase in fluorescence quantum yield. However, further work is needed to discern changes in the radiative and non-radiative decay rates caused by coupling to the plasmonic modes in the nanostructured Au/Au film. 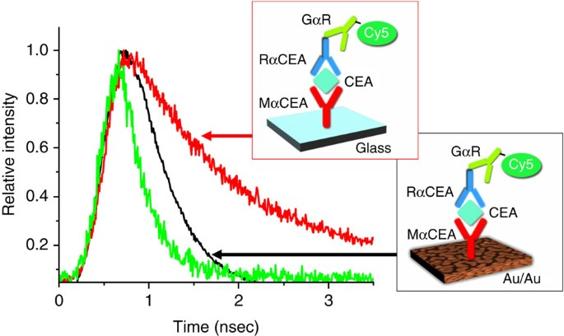Figure 3: Fluorescence lifetime measurements on protein microarrays. Ensemble fluorescence decay of goat anti-rabbit IgG-Cy5 labelling a CEA assay (100 pM analyte concentration) on an Au/Au film (black line) or glass slide (red line), diagrammed in schematic at right. The excited state lifetime of the Cy5 fluorophore is greatly reduced in proximity to the Au/Au film compared with glass, likely resulting in an increased apparent quantum yield. The instrument response function is shown in green. Figure 3: Fluorescence lifetime measurements on protein microarrays. Ensemble fluorescence decay of goat anti-rabbit IgG-Cy5 labelling a CEA assay (100 pM analyte concentration) on an Au/Au film (black line) or glass slide (red line), diagrammed in schematic at right. The excited state lifetime of the Cy5 fluorophore is greatly reduced in proximity to the Au/Au film compared with glass, likely resulting in an increased apparent quantum yield. The instrument response function is shown in green. Full size image μArray/Au detection of biomarkers in xenograft mouse serum To demonstrate the utility of NIR-FE protein microarrays, detection of serum cancer biomarkers was conducted by preparing mouse models bearing xenograft tumours of the LS174T colon cancer model, known to over-express and shed CEA into the bloodstream [23] . Two million LS174T cells per xenograft were inoculated subcutaneously into athymic nude mice and allowed to grow over the course of three weeks. Blood samples were extracted from the tail before inoculation, as well as at several time points during the course of tumour growth, with serum samples isolated by centrifugation (see Methods). Tenfold dilution of just 2 μl of sample serum allowed quantification of serum CEA levels on μArray/Au against a standard curve, obtained with calibration spots (assay spots exposed to known CEA concentrations) on the same μArray/Au substrate ( Fig. 4a,b ). Two mouse models were prepared for this study, and their serum CEA levels were analysed in separate experiments on μArray/Au assays labelled by IR800. In comparison to calibration curves, serum samples taken before inoculation of LS174T indicated no measurable CEA; however, detectable levels of CEA were observed in both mice when the xenograft tumour volume reached ∼ 30–50 mm 3 ( Fig. 4 ). 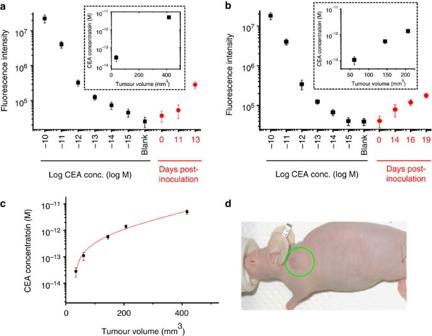Figure 4: μArray/Au measurement of CEA in the sera of LS174T xenograft tumour mouse models. (a) CEA calibration curve (black squares) measured from a μArray/Au assay labelled by goat anti-rabbit IgG-IR800 conjugates along with the tenfold diluted serum of a xenograft mouse model bearing an LS174T tumour at different post-inoculation time points (red circles). Dilution of sera is necessary due to low volume of tail-extracted blood samples. Actual blood pool CEA concentrations are calculated by comparison of diluted serum sample fluorescence intensity to a sigmoidal fit of the accompanying calibration curve, followed by correction for dilution (tenfold). Calibration curves in this case and in (b) were obtained by spiking known concentrations of CEA into tenfold diluted normal mouse serum (b) An additional data set as described in (a) performed on a different μArray/Au assay substrate with serum from a different LS174T tumour-bearing mouse and a uniquely generated calibration curve. Insets in (a) and (b) relate tumour volume with dilution-corrected CEA serum concentrations. In each case, a calibration curve is performed on the same μArray/Au assay substrate as the mouse serum sample measurements to account for slight variations from slide to slide in Au/Au film preparation and robotic printing of capture antibody. (c) Combination of the LS174T xenograft mouse model data (a) and (b) showing similar growth behaviour. The relation between LS174T tumour volume and increase in CEA serum concentration is well fit by an exponential growth curve (red line). (d) Representative photographic image of a nude mouse bearing an LS174T xenograft tumour (green circle). Figure 4: μArray/Au measurement of CEA in the sera of LS174T xenograft tumour mouse models. ( a ) CEA calibration curve (black squares) measured from a μArray/Au assay labelled by goat anti-rabbit IgG-IR800 conjugates along with the tenfold diluted serum of a xenograft mouse model bearing an LS174T tumour at different post-inoculation time points (red circles). Dilution of sera is necessary due to low volume of tail-extracted blood samples. Actual blood pool CEA concentrations are calculated by comparison of diluted serum sample fluorescence intensity to a sigmoidal fit of the accompanying calibration curve, followed by correction for dilution (tenfold). Calibration curves in this case and in ( b ) were obtained by spiking known concentrations of CEA into tenfold diluted normal mouse serum ( b ) An additional data set as described in ( a ) performed on a different μArray/Au assay substrate with serum from a different LS174T tumour-bearing mouse and a uniquely generated calibration curve. Insets in ( a ) and ( b ) relate tumour volume with dilution-corrected CEA serum concentrations. In each case, a calibration curve is performed on the same μArray/Au assay substrate as the mouse serum sample measurements to account for slight variations from slide to slide in Au/Au film preparation and robotic printing of capture antibody. ( c ) Combination of the LS174T xenograft mouse model data ( a ) and ( b ) showing similar growth behaviour. The relation between LS174T tumour volume and increase in CEA serum concentration is well fit by an exponential growth curve (red line). ( d ) Representative photographic image of a nude mouse bearing an LS174T xenograft tumour (green circle). Full size image We observed a clear increase in CEA serum concentration with increasing tumour volume. Sera sampled following LS174T inoculation yielded CEA blood pool concentrations ranging from ∼ 30 fM up to 5 pM with tumour volumes ranging from ∼ 35 mm 3 to 425 mm 3 ( Fig. 4a–c ). Under the tenfold serum sample dilution conditions used in our μArray/Au assays, all serum samples contained CEA at levels undetectable by conventional ELISA, which possesses a limit of detection between 1 and 5 pM. A plot of CEA serum concentrations versus tumour volume demonstrated an exponential growth behaviour ( Fig. 4c ), suggesting that the mouse model serum CEA levels change rapidly during the initial phase of tumour growth. Multiplexed μArray/Au assays for autoantibody detection The multiplex capabilities and small sample volume requirements of planar protein microarrays afford a wealth of information regarding both proven and putative protein biomarkers. Autoantigen microarrays have demonstrated utility in proteomic analysis of various human autoimmune disease processes and led towards improved diagnostic tests and a greater understanding of the underlying disease pathophysiology [4] . To explore the multiplex capabilities of μArray/Au assays, we printed a total of 32 analytes in triplicate, including human autoantigens and controls ( Supplementary Table S1 ) onto μArray/Au, commercial nitrocellulose, and glass substrates. The resulting autoantigen array was incubated with a mixture of human sera, containing both characterized autoantibodies with reactivity towards several autoantigen targets as well as poorly characterized antibodies with unknown reactivities (Methods), at 1:300 dilution, and probed with IR800-conjugated goat anti-human IgG. The arrays were scanned and analysed using commercially available equipment and software (Methods). Compared with both highly porous nitrocellulose and planar glass substrates, our autoantigen μArray/Au afforded increased feature intensities owing to NIR-FE ( Fig. 5 ). Notably, the high background intensity of nitrocellulose was a result of the combined effects of autofluorescence and nonspecific binding. Background intensity of μArray/Au substrates and glass under 785 nm excitation were approximately tenfold lower than nitrocellulose. On nitrocellulose films, the 32-autoantigen array showed intensities spanning merely half of an order of magnitude, whereas the same array formed on gold exhibited intensities spanning two orders of magnitude ( Fig. 5b ). The autoantigen microarray intensities of μArray/Au were 25–50 times higher than on glass. Clearly, the NIR fluorescence enhancement and reduced background afforded by the multiplexed μArray/Au assay afforded increased sensitivity for autoantibody reactivity and broadened dynamic range ( Fig. 5b ). 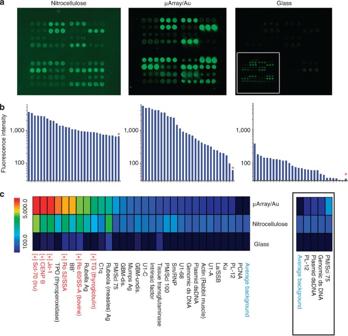Figure 5: Multiplexed autoantigen arrays probed with human serum containing autoantibodies. (a) Fluorescence intensity maps generated by scanning IR800-labelled autoantigen/autoantibody arrays, on nitrocellulose, μArray/Au, and glass, with the Licor Odyssey in the 800 nm channel. All images are shown on the same intensity scale, while the scale of the inset in the fluorescence intensity map of glass is increased tenfold. (b) Log scale plot of mean pixel intensity of autoantigen/autoantibody features and average background (denoted by red asterisk) for features printed in triplicate. (c) Intensity heatmap comparing the mean feature intensities of the same autoantigens on μArray/Au, nitrocellulose, and glass. '[+]' indicates autoantigens with characterized positive reactivity towards components of the autoimmune serum mixture, shown in red. The simplified heatmap (right, boxed) with identical intensity scale shows only those antigens with low but significant intensity on μArray/Au, yet appear no different than background on nitrocellulose and glass, as described in the text. SeeSupplementary Table S1for autoantigen print layout and a description of each autoantigen. Figure 5: Multiplexed autoantigen arrays probed with human serum containing autoantibodies. ( a ) Fluorescence intensity maps generated by scanning IR800-labelled autoantigen/autoantibody arrays, on nitrocellulose, μArray/Au, and glass, with the Licor Odyssey in the 800 nm channel. All images are shown on the same intensity scale, while the scale of the inset in the fluorescence intensity map of glass is increased tenfold. ( b ) Log scale plot of mean pixel intensity of autoantigen/autoantibody features and average background (denoted by red asterisk) for features printed in triplicate. ( c ) Intensity heatmap comparing the mean feature intensities of the same autoantigens on μArray/Au, nitrocellulose, and glass. '[+]' indicates autoantigens with characterized positive reactivity towards components of the autoimmune serum mixture, shown in red. The simplified heatmap (right, boxed) with identical intensity scale shows only those antigens with low but significant intensity on μArray/Au, yet appear no different than background on nitrocellulose and glass, as described in the text. See Supplementary Table S1 for autoantigen print layout and a description of each autoantigen. Full size image Good agreement in autoantigen-antibody reactivity was observed between the three assay substrates; however, features on glass often failed to provide sufficient signal-to-background for quantification ( Fig. 5c ). The incubated serum mixture (Methods) contained characterized human autoantibodies against SS-A, Jo-1, centromere protein B, thyroglobulin, and DNA topoisomerase-1 (scl-70, truncated fragment), all of which were detected with high intensity as expected on their conjugate antigen feature ( Supplementary Table S1 ). Several other autoantigen features on μArray/Au, but not on nitrocellulose or glass substrates, could be easily distinguished from background with significant signal-to-background ratios ( Fig. 5c ). The sera sample was not known or characterized to exhibit reactivity towards these autoantigens [24] . Our simple and scalable solution-phase growth methodology affords uniform, plasmonic, nanostructured gold films on glass slides, capable of intensifying the emission of near-infrared fluorophores. Fluorescence enhancement is found to be dependent on plasmon resonance, gold film structure, and the fluorophores used to probe the fluorescence enhancement phenomenon. Employment of μArray/Au assays for quantification of protein biomarkers results in significantly improved detection limits and broader dynamic ranges than traditional protein microarrays and ELISA. Moreover, multiplexed protein microarrays performed on μArray/Au benefit from enhanced feature intensity and low-autofluorescence background, compared with commercially available glass and nitrocellulose substrates, thus providing a broader dynamic range with increased sensitivity for protein microarrays. Excitation field enhancement, resulting in an increased optical transition rate, is believed to be a contributing factor to our observations of NIR-FE [20] , [21] . Previous results suggest that excitation field enhancement is strongest within the gaps of the gold island structure of Au/Au films [17] . In this study, we found that optimal NIR-FE is provided by Au/Au films containing dense gold islands with an average inter-island gap distance of ∼ 36 nm. On the other hand, thick Au/Au films containing a semi-continuous layer of gold (few gaps present) yielded little fluorescence enhancement relative to a bare glass substrate, whereas completely continuous gold films (no gaps present) resulted in quenching of fluorescence. We therefore attribute the nanoscale gaps in our Au/Au films, and the resulting enhanced excitation electric fields, as one of the causes of fluorescence enhancement on our μArray/Au platform [20] . Proximity of a fluorophore to a metal structure could quench fluorescence emission due to a greater enhancement of the non-radiative decay rate k nr than the radiative decay rate k rad (refs 13 , 25 , 26 ). Fluorophore coupling to the scattering component of plasmonic extinction is responsible for increased radiative decay rates resulting in fluorescence enhancement, whereas the absorption component is responsible for enhancing the rate of non-radiative decay and thus fluorescence quenching [15] . The magnitude of absorption and scattering components of the optical spectra of metal nanoparticles depends on both the size and shape of the metal structures, as described by Mie theory [13] , [26] . Significantly increased non-radiative decay rates could be the cause of fluorescence quenching, rather than enhancement, on continuous films. The scattering (re-radiating) efficiency of our Au/Au film for fluorescence enhancement is large in the near-infrared where the plasmonic peaks of the Au/Au films overlap with the fluorescence emission wavelengths of the IR800 and Cy5 fluorophores. The plasmonic resonance peaks of our Au/Au films reside in this NIR region due to the wavelength-dependent dielectric constant of gold, suitable sizes of the gold islands, and possibly the elongated shapes of the islands [13] , [27] in the Au/Au films. We attribute NIR-FE of IR800 and Cy5 labels in our μArray/Au to the optimal gold island size (on the order of 10 4 nm 2 ) and the coupling of the dipolar components of the plasmonic modes of these nanoislands to the emission of fluorescence. The suitable Au islands sizes and plasmonic coupling in these nanostructured Au/Au films may have led to an increase in k rad that outweighed k nr enhancement of the near-infrared fluorophores used herein for microarray protein assays, contributing to an increased apparent quantum yield and improved signal-to-noise ratios for protein detection. Further research into the effect of our nanostructured Au/Au film on radiative and non-radiative decay rates of IR800 and Cy5 is underway. The observed variation in enhancement factor between Cy5 and IR800 on a given Au/Au film is likely due to several contributing factors. First, because the observed quantum yield scales with the ratio of radiative decay rate to total decay rate, the radiative decay rate could be enhanced relatively more than the non-radiative decay rate for inherently low quantum yield emitters [12] (η ∼ 7% for IR800 versus ∼ 20% for Cy5). Also, the different excitation and emission energies of the fluorophores may interact differently with absorbance and scattering components of an Au/Au film with fixed plasmon resonance. It is presumed that only the scattering component of metal nanoparticles contributes to far field radiation [10] , which is greater at longer wavelengths, such as those characteristic of IR800. Finally, the incident field enhancement efficiency of metal nanostructures is dependent on both nanoparticle spacing as well as wavelength. Peak field enhancements are obtained at longer wavelengths when nanoparticle separation distances are small [28] . Combined with the benefit of low biological autofluorescence in the near-infrared excitation/emission region and increased surface area, the improved signal-to-noise ratios of μArray/Au assays provide vastly improved sensitivity for quantification of disease biomarkers in biological media. Unlike chemical amplification methods, metal-enhancement of NIR fluorescence emission increases signal without creating undesirable background or extra noise. μArray/Au assays afford increased signal-to-noise ratios by ∼ 15-fold for Cy5-labelled sandwich assays and ∼ 100-fold for IR800-labelled sandwich assays relative to identical protein microarray sandwich assays on glass slides. The fivefold increase in fluorescence enhancement for Cy5 and IR800 employed in immunoassay experiments compared with drop-dried samples is probably caused by alleviation of non-radiative energy transfer to the metallic film at greater separation distances, in agreement with previous literature [29] . For detection and quantification of CEA spiked into 100% serum, such gains in signal-to-noise resulted in improved detection limits to 5 fM with a dynamic range over six orders of magnitude. Detection of CEA in the serum of xenograft mouse models bearing LS174T tumours was accomplished by use of μArray/Au assays. In comparison to a calibration curve, serum CEA concentrations in the range of ∼ 30 fM to 100 fM were detectable when tumour volumes were well below 100 mm 3 . We note that with detection limits in the range of 1–5 pM, commercially available CEA ELISA kits fail to provide adequate sensitivity to detect or quantify CEA in the majority of the ex vivo serum samples analysed in the present study. Moreover, protein diagnostics based on highly sensitive μArray/Au assays require far less sample volume than ELISA and may be multiplexed to analyse a variety of protein biomarkers at once. To demonstrate the multiplexing capabilities of μArray/Au substrates, a panel of human autoantigens was printed onto μArray/Au substrates, as well as commercially available nitrocellulose membrane substrates and glass slides. The autoantigens printed represent both well-characterized and poorly characterized targets of human autoantibodies implicated in a range of autoimmune diseases including systemic lupus erythematosus (SLE), Sjögren syndrome, mixed connective tissue disease, systemic sclerosis, celiac disease, Goodpasture's syndrome, and others [4] , [30] , [31] , [32] , [33] . Incubation of a mixture of human sera (Methods) containing known reactivity towards several autoantigen targets led to the observation of a broad range of reactivities, represented as microarray feature intensities, with which the various assay substrates could be compared and contrasted. Nitrocellulose-based substrates were often used for protein microarrays, because they provide a high-surface area, 11 μm thick, three-dimensional polymer layer for capture reagent immobilization, with a protein binding capacity [34] of ∼ 4,000 ng mm −3 . In contrast, planar surfaces, such as μArray/Au and glass, provide binding capacities in the range of 10–100 ng mm −2 . Therefore, protein microarrays, such as autoantigen arrays, on nitrocellulose membranes yield high feature intensities through increased capture efficiency (vide supra). On the other hand, nitrocellulose films are known to exhibit high autofluorescence in the visible, limiting their dynamic range and utility. Autofluorescence of nitrocellulose is mitigated to an extent by employing fluorescence excitation and emission energies in the near-infrared (for example, Cy5 and IR800 dyes); however, we have observed that sufficient background intensity remains, even at emission wavelengths from 700–800 nm emission ( Fig. 5 ; Supplementary Fig. S11 ), to prevent identification of dilute or low-reactivity autoantibodies. The dynamic range of this IR800-labelled autoantigen array on nitrocellulose was half-an-order of magnitude, whereas the background intensity and maximum observed feature intensity of an autoantigen array labelled by Cy5 differed only by a factor of 2. In contrast, μArray/Au substrates afford higher positive signals owing to fluorescence enhancement as well as tenfold lower autofluorescence backgrounds compared with nitrocellulose. With a much broader fluorescence intensity range ( ∼ 2 orders of magnitude) than nitrocellulose ( ∼ half of an order of magnitude) in this multiplexed autoantigen array, μArray/Au substrates identified not only the highly reactive autoantibodies in the serum mixture, but also other autoantigen features with non-negligible reactivity towards the antoantibody-containing serum ( Fig. 5a,c ). μArray/Au also outperformed planar glass substrates, with vastly increased positive intensities and higher signal-to-noise ratios owing to NIR-FE. All assay substrates exhibited positive feature intensities for highly reactive markers of autoimmune conditions such as Lupus (for example, SLE, and subacute cutaneous lupus erythematosus, SCLE), Sjögren Syndrome, systemic sclerosis, poly- and dermato-myositis, and thyroiditis. The sample of mixed autoimmune serum employed here included well-characterized [4] , [24] autoantibodies targeting Ro/SS-A, Jo-1, centromere protein B, thyroglobulin and DNA topoisomerase-1 (scl-70), all of which were detected with high intensity as expected on their conjugate antigen feature. The serum sample also contains autoantibodies towards myeloperoxidase, proteinase 3, histones, and mitrochondrial antigen, which were not included in the autoantigen array. Moreover, it is expected that the serum mixture also includes uncharacterized autoantibodies and other human immunoglobulin Gs that may contribute to intermediate and low levels of array feature intensity. For example, non-negligible intensity was observed on both nitrocellulose and μArray/Au representing reactivity of the serum mixture towards thyroperoxidase, Sm protein B/B', measles antigen, glomerular basement membrane antigen, complement complex C1q, and components of the U1-snRNP complex (for example, U1-C, U1-A, sm/RNP). Autoantibodies of PCNA, implicated in SLE, were not observed on any of the substrates tested. However, the μArray/Au substrate revealed slight reactivity, not known a priori, of the incubated autoimmune sera towards autoantigens including double-stranded DNA, PL-12, and PM/Scl-75 ( Fig. 5c ), which, on nitrocellulose, did not present feature intensity of significant difference from the background. These antigens are implicated in autoimmune disorders such as SLE, polymyositis, and polymyositis-systemic sclerosis overlap syndrome, respectively. Our results suggest that in addition to improved detection limits for protein-based diagnostics (for example, early cancer detection), μArray/Au protein assays could significantly enhance our ability to elucidate intermediate and low-level autoantibody reactivity in autoimmune diseases. In general, the higher sensitivity and broader dynamic range afforded by μArray/Au substrates will benefit high-throughput proteomics research, as well as diagnostics, for a wide range of diseases throughout various biological fields. In conclusion, μArray/Au assays afford a significant improvement in signal-to-noise ratio, resulting in multiplexed microarray protein sandwich assays possessing a broad dynamic range and high sensitivity, with detection limits ∼ 1,000 to 5,000-fold lower than traditional techniques, yet they require no additional assay steps and are compatible with standard protein microarray processing and equipment. The NIR-FE μArray/Au assays rely on physical principles, namely an enhancement in excitation field strength, reduction in excited state lifetime, and overall apparent increase in fluorescence quantum yield, to significantly improve the signal-to-noise ratio over standard protein microarrays. Our solution phase, bottom-up growth procedure of Au/Au films for fluorescence enhancement applications is scalable, simple and fast. The Au/Au film substrates for NIR-FE applications are stable over time and in biological media, and, moreover, are uniform enough to provide quantitative analysis with a dynamic range of over six orders of magnitude. In addition to affording biomarker quantification at low concentrations, high-throughput screening methods may benefit from the expanded dynamic range afforded by multiplexed μArray/Au assays, where concentrations of analytes, as well as binding constants, may span a significant and unknown range. NIR-FE based on Au/Au films may also find further applications as an in vitro imaging tool. For example, fluorescent agents bound to the membrane of live cells have been enhanced by Au/Au films [35] . Coupled with the simplicity afforded by physical signal enhancement and compatibility with existing microarray tools, μArray/Au assays are expected to find broad use in disease diagnosis and protein biomarker discovery applications. Conjugation of IR800 to goat anti-rabbit IgG IR800cw-NHS ester was dissolved in dry DMSO. IR800cw-NHS ester was mixed with goat anti-rabbit IgG in PBS at a 4:1 mole ratio and incubated in the dark at room temperature for 1 h following excess removal by G-25 NAP-5 columns, resulting in a loading of ∼ 1 dye per IgG. Preparation of gold-on-gold (Au/Au) films Gold-on-gold (Au/Au) films were prepared [17] by immersing a glass slide into a solution of 3 mM HAuCl 4 (aq). 20 μl of NH 4 OH was added per ml of total volume with rapid shaking for one minute. The substrate was submerged in two clean water baths to remove unbound Au 3+ precipitate and then was immersed into 1 mM NaBH 4 for 1 min, which completed the seeding step. After washing, the substrate was immersed into a 1:1 aqueous solution of HAuCl 4 and NH 2 OH (for example, 750 μM) and uniformly shaken for 5 min, followed by a 10-min incubation to complete the growth step. The substrate was washed again by immersion into water and blown dry. The plasmon resonance of the resulting Au/Au films was measured using a Cary 300 UV-vis-NIR absorbance spectrometer after correcting for background absorbance from the glass substrate. Scanning electron micrographs were acquired on an FEI XL30 Sirion SEM with FEG source at 5 kV acceleration voltage. Attachment of 6PEG-COOH to films and microarray printing Au/Au substrates were immersed into 10 mM cysteamine in ethanol overnight at room temperature. After rinsing with ethanol and drying, the amine-functionalized Au/Au substrate was immersed in a solution of 20 μM 6-arm poly(ethylene glycol)-carboxylate ( M n ∼ 10,000 Da) and 20 mM each of 1-ethyl-3-(3-dimethylaminopropyl) carbodiimide and N -hydroxysuccinimide (NHS) in dimethylformamide (DMF). After rinsing the Au/Au substrate with ethanol and drying, NHS-activated Au/Au and bare glass substrates were loaded into a microarray printing robot where 5 μM monoclonal mouse anti-CEA IgG in PBS supplemented with 0.1% glycerol and 0.01% tween-20 was printed via solid pins at 25 °C and 65% humidity, resulting in microarray feature diameters of ∼ 400 μm, printed into 12 sets of 12 spots. The slides were dried with compressed air and blocked shortly after printing. For preparation of autoantigen arrays, functionalized Au/Au films, glass slides and two-pad nitrocellulose slides were loaded into a microarray robot contact printer at 25 °C and 65% humidity. Autoantigens purchased from Diarect, Molecular Probes, Biodesign, Immunovision, or Sigma-Aldrich (see Supplementary Methods ) were printed in triplicate in PBS supplemented with 0.01% tween-20 and glycerol at the concentrations and in the order indicated in Supplementary Table S1 . Microarray CEA sandwich assay procedure See Supplementary Methods for a detailed description of the microarray protein sandwich assay procedure. Briefly, slides were blocked overnight at 4 °C in a solution containing 3% fetal bovine serum (FBS) in PBS containing 0.05% tween-20 (PBST). Purified CEA was diluted into pure FBS, and 20 μl of each CEA solution (CEA concentrations varied from 1 nM to 1 fM) was applied to each set of spots along with a control of only pure FBS (blank) and incubated 6 h at room temperature, followed by washing. Polyclonal rabbit anti-CEA was incubated over each set of array spots at 10 nM in PBS and incubated at room temperature in a humid environment for 1.5 h. Assays were again washed and 500 pM of Cy5 or IR800-conjugated polyclonal goat anti-rabbit IgG was incubated for 10 min at room temperature. Assay substrates were washed three times in PBST and once in PBS, followed by immersion in deionized water and were subsequently blown dry with compressed air. When xenograft serum samples were to be included along with a calibration curve, purified CEA was diluted into 10% normal mouse serum supplemented with 3% FBS in PBS rather than pure FBS, and 2 μl of xenograft serum was diluted to 20 μl by 3% FBS in PBS. All other steps remain the same. The resulting tenfold diluted xenograft CEA serum fluorescence intensities were compared with a sigmoidal fit of the accompanying calibration curve and then corrected for the tenfold dilution to calculate the original serum concentration. Multiplexed autoantigen microarray assay procedure Autoantigen arrays ( Supplementary Table S1 ) on μArray/Au, nitrocellulose and Superfrost Plus glass substrates were blocked overnight at 4 °C in a solution containing 3% FBS in PBST. An equivolume mixture of reactive human sera [24] (Immunovision, used as received), containing characterized autoantibodies against Smith antigen, SS-A antigen, centromere antigen, Ribosomal P antigen, histones, thyroglobulin, myeloperoxidase, proteinase 3, topoisomerase I, mitochondrial antigen and Jo-1 (included at 0.75 equivalent fractional volume), was diluted 1:300 in 10% FBS and incubated on the autoantigen arrays for 3 h at room temperature, followed by washing with PBST. Subsequently the array was probed with goat anti-human IgG secondary antibody labelled with IR800 at 1 nM ( ∼ 1 dye/antibody) in 10% FBS in PBST for 10 min at room temperature. Assay substrates were washed three times in PBST and once in PBS, followed by immersion in deionized water and were subsequently blown dry with compressed air. Fluorescence measurement and analysis A Horiba Jobin Yvon Labram HR800 confocal laser scanning microscope was used for the majority of fluorescence measurements presented herein. See Supplementary Methods for detailed description of the setup and measurement conditions. Horiba Jobin Yvon Labspec software, or occasionally GenePix 6.0 (Molecular Devices), was used to analyse and quantify fluorescence emission. Using Labspec, the average local background was subtracted and the average spectrum for each array feature or protein spot was averaged. Standard deviations represent the standard error of the means of twelve replicate spot features for each CEA concentration. Fluorescence was quantified by integrating the baseline-corrected, fluorescence emission peak (645–740 nm for Cy5 and 790875 nm for IR800). The Molecular Devices Genepix 4000B Axon scanner and Licor Odyssey scanner were also used to verify compatibility of μArray/Au assays with commercial systems. Multiplexed autoantigen/autoantibody arrays were scanned using the Licor Odyssey Scanner, 800 nm channel with gain set to 6.0, 42 μm. Genepix 6.1 was used to automatically identify features above composite pixel intensity of 5. Fluorescence intensities presented in Figure 5b are the average of mean pixel intensity values for features printed in triplicate. Fluorescence lifetime measurement Fluorescence lifetimes of Cy5 and IR800 conjugated to IgG molecules were measured by time-correlated single photon counting (TCSPC). For sandwich assay lifetime measurements, a CEA sandwich assay was performed as described above on an Au/Au film, as well as on a borosilicate glass coverslip. See Supplementary Methods for a detailed description of the TCSPC setup and analysis. Xenograft models and animal handling Athymic nude female mice obtained from Charles River were housed at Stanford Research Animal Facility under Stanford Institutional Animal Care and Use Committee protocols. When the mice reached 8 weeks in age, they were inoculated with 2 million LS174T cells subcutaneously on the shoulder. At the given time points, ∼ 100 μl of blood was collected from the tail of the mice. The blood was then centrifuged at 10,000 g for 20 min to fractionate the blood and collect the serum. During the tumour inoculation and blood collection, the mice were anaesthesized by inhalation of 2% isoflurane mixed with oxygen accordingly to an approved animal protocol. The tumour width and length was measured using a digital caliper. The tumour volume was derived from the modified ellipsoidal formula: Volume = (Width×Width×Length)/2. How to cite this article: Tabakman, S. M. et al . Plasmonic substrates for multiplexed protein microarrays with femtomolar sensitivity and broad dynamic range. Nat. Commun. 2:466 doi: 10.1038/ncomms1477 (2011).